Helicobacter pyloriCagA promotes Snail-mediated epithelial–mesenchymal transition by reducing GSK-3 activity Cytotoxin-associated gene A (CagA) is an oncoprotein and a major virulence factor of H. pylori . CagA is delivered into gastric epithelial cells via a type IV secretion system and causes cellular transformation. The loss of epithelial adhesion that accompanies the epithelial–mesenchymal transition (EMT) is a hallmark of gastric cancer. Although CagA is a causal factor in gastric cancer, the link between CagA and the associated EMT has not been elucidated. Here, we show that CagA induces the EMT by stabilizing Snail, a transcriptional repressor of E-cadherin expression. Mechanistically we show that CagA binds GSK-3 in a manner similar to Axin and causes it to shift to an insoluble fraction, resulting in reduced GSK-3 activity. We also find that the level of Snail protein is increased in H. pylori infected epithelium in clinical samples. These results suggest that H. pylori CagA acts as a pathogenic scaffold protein that induces a Snail-mediated EMT via the depletion of GSK-3. Gram-negative bacterium Helicobacter pylori ( H. pylori ) is the major pathogenic microorganism of human stomach, responsible for a wide range of disorders, from chronic gastritis to gastric cancer [1] , [2] . A major virulence factor of H. pylori , CagA (cytotoxin-associated gene A) protein is delivered into the gastric epithelial cells through a bacterial type IV secretion system and plays a critical role in cell transformation [3] , [4] . In this process, CagA undergoes tyrosine phosphorylation by Src family kinases or c-Abl kinase at the repeated Glu-Pro-Ile-Tyr-Ala (EPIYA) motifs followed by binding to SHP2 tyrosine phosphatase [5] , [6] . CagA binds to and activates/inactivates multiple signalling proteins in an EPIYA motif phosphorylation-dependent or -independent manner, influencing actin-cytoskeletal rearrangements and the disruption of cell-to-cell junctions as well as proliferative, proinflammatory and antiapoptotic nuclear responses [7] . The EPIYA phosphorylation status of CagA also affects the signal switch between the SHP2/ERK and JAK/STAT3 pathways via gp130 in gastric epithelial cells [8] . While the causality of CagA on gastric cancer has been clearly demonstrated in vivo [9] and several membranous targets of CagA, such as gp130 and PAR1, have been identified [8] , [10] , the molecular mechanism by which intracellular target of CagA results in cellular transformation and carcinogenesis has not been fully elucidated. The epithelial–mesenchymal transition (EMT) is a complex cellular programme involved in both development and cancer, its hallmark being the loss of cell–cell adhesion [11] , [12] . While the loss of epithelial adhesion is known for its critical role in the metastatic progression of cancer, it is also a well-established genetic background of hereditary gastric carcinoma accompanying germ-line mutation of E-cadherin [13] . Furthermore, an exome sequencing study has revealed that loss of cell adhesion by somatic mutation constitutes a genetic background of sporadic gastric cancer [14] . The zinc-finger transcription factor Snail has been implicated in E-cadherin suppression via its binding to E-cadherin proximal promoter [15] . As the destruction box on β-catenin ( CTNNB 1) is regulated by Wnt signalling, the Snail harbours similar canonical GSK-3 destruction motifs wherein Wnt signalling or hyperglycemic condition stabilizes Snail protein in the same manner through inhibition of serial phosphorylation by GSK-3 (refs 16 , 17 ). During the signal transduction of the Wnt cascade, the scaffolding protein Axin plays a key role by binding to GSK-3 (refs 18 , 19 ). Specifically, the nuclear export function of Axin2 serves as a nuclear–cytoplasmic shuttle for GSK-3, resulting in the stabilization of nuclear Snail and inducing the EMT programme of cancer cells [20] . Recently, the tumour suppressor p53/miRNA-34 axis has been identified as regulating embryonic development and carcinogenic progression through the post-transcriptional repression of a set of genes involving Wnt signalling and the EMT programme in parallel [21] , [22] , [23] . The CagA-induced cellular transformation associated with cell motility and scattering, known as the ‘hummingbird phenotype’, has been well described [24] . In this study, we report that CagA accelerates Snail-mediated EMT on gastric epithelial cells by depleting endogenous GSK-3, a consequence similar to canonical Wnt activation. Mechanistically, the CagA depletes the endogenous GSK-3, causing its transition to insoluble fraction and subsequent suppression of endogenous kinase activity. Interestingly, the suppression of GSK-3 by CagA also regulates protein abundance of another GSK-3 substrate, MCL-1, and active AMP-activated protein kinase (AMPK), indicating that GSK-3 depletion by H. pylori may have a wider role in oncogenic pathways, beyond the Snail-mediated EMT process. H. pylori induces EMT in a CagA-dependent manner H. pylori induces an elongated ‘hummingbird phenotype’ with the loss of epithelial polarity and stimulates epithelial cell migration [10] , [25] . To examine whether CagA translocation by H. pylori infection induces EMT with loss of E-cadherin, we infected gastric cancer cells with bacterial strain 60190 (CagA-positive H. pylori ) or transfected them with CagA expression vectors. Treatment with 60190 or overexpression of CagA suppressed the abundance of membrane-localized E-cadherin in gastric cancer cells with increased Tyr phosphorylation ( Fig. 1a ). Because H. pylori infection and CagA translocation promote EMT [26] , we re-evaluated the capacity of our bacterial strain and expression vector to increase cell migration potential. The cell motilities on scratch wound or transwell migration significantly increased on 60190 infection or CagA expression vector while isogenic mutant strain of 60190 lacking CagA did not ( Fig. 1b and Supplementary Fig. 1 ). CagA was also functional in inducing in vivo invasive progression of non-invasive MCF-7 cells, as seen in the crossing of cells into the basement membrane in the chick chorioallantoic membrane (CAM) assay ( Fig. 1c ). 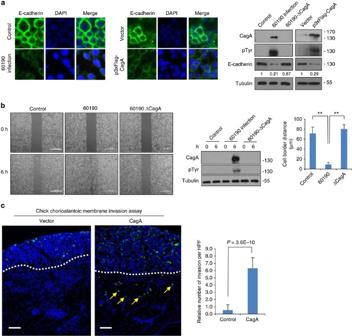Figure 1:H. pyloriinduces CagA-dependent EMT in gastric cancer cells. (a) E-cadherin expressions in MKN28 gastric cancer cells infected with CagA-positive 60190 (left panels) or transfection of CagA expression vector (middle panels) were assessed by indirect immunofluorescence with anti-E-cadherin antibody (green) and 4',6-diamidino-2-phenylindole (DAPI) nuclear stain (blue). Following infection or transfection, the protein abundances of CagA, phospho-Tyr (pTyr) and E-cadherin were assessed by immunoblot analysis (right panels). Tubulin was used as the loading control; relative abundance of each loading control is denoted below the blot. (b) Confluent AGS cells were wounded and then infected with 60190 or isogenic CagA deletion mutant strain for 6 h (left panels). Protein lysates from AGS cells of the migration assay were analysed by immunoblotting for CagA translocation and pTyr (middle panels). Distance between the cell borders was measured from five independent sites after 6 h infection (right panel, **P<0.01 by Student’st-test). Error bars indicate s.d. Scale bar, 100 μm. (c) The non-invasive MCF-7 cells were transiently co-transfected with either a control or CagA with GFP expression vector. The cells were cultured atop the embryonic chick chorioallantoic membrane (CAM) for 3 days and the fixed tissue sections then were examined by fluorescence microscopy. The upper face of the CAM is indicated by dashed white lines; invasive cancer cells are denoted by arrows. Scale bars, 300 μm. The number of GFP-positive invasive cells under the basement membrane were quantitated and statistically analysed by Student’st-test (right panel). Error bars indicate s.d. Figure 1: H. pylori induces CagA-dependent EMT in gastric cancer cells. ( a ) E-cadherin expressions in MKN28 gastric cancer cells infected with CagA-positive 60190 (left panels) or transfection of CagA expression vector (middle panels) were assessed by indirect immunofluorescence with anti-E-cadherin antibody (green) and 4',6-diamidino-2-phenylindole (DAPI) nuclear stain (blue). Following infection or transfection, the protein abundances of CagA, phospho-Tyr (pTyr) and E-cadherin were assessed by immunoblot analysis (right panels). Tubulin was used as the loading control; relative abundance of each loading control is denoted below the blot. ( b ) Confluent AGS cells were wounded and then infected with 60190 or isogenic CagA deletion mutant strain for 6 h (left panels). Protein lysates from AGS cells of the migration assay were analysed by immunoblotting for CagA translocation and pTyr (middle panels). Distance between the cell borders was measured from five independent sites after 6 h infection (right panel, ** P <0.01 by Student’s t -test). Error bars indicate s.d. Scale bar, 100 μm. ( c ) The non-invasive MCF-7 cells were transiently co-transfected with either a control or CagA with GFP expression vector. The cells were cultured atop the embryonic chick chorioallantoic membrane (CAM) for 3 days and the fixed tissue sections then were examined by fluorescence microscopy. The upper face of the CAM is indicated by dashed white lines; invasive cancer cells are denoted by arrows. Scale bars, 300 μm. The number of GFP-positive invasive cells under the basement membrane were quantitated and statistically analysed by Student’s t -test (right panel). Error bars indicate s.d. Full size image CagA promotes EMT by stabilizing Snail protein The potent E-cadherin repressor Snail has been proposed to have important functions in carcinogenesis and cancer progression through its role in EMT [27] , [28] . To test whether Snail protein abundance in gastric cancer cells was responsible for CagA-dependent EMT, AGS and MKN28 gastric cancer cells were infected with the 60190 strain and an isogenic strain lacking CagA or transfected by CagA expression vector. Indeed, H. pylori inducing wild-type (wt) CagA or CagA expression vector increased endogenous Snail protein abundance in a time-dependent manner, whereas the strain lacking CagA did not ( Fig. 2a and Supplementary Fig. 2a ). As Snail is well known to suppress E-cadherin [15] , [17] , both E-cadherin promoter activities and mRNA transcript levels were repressed in CagA-dependent manner ( Fig. 2b and Supplementary Fig. 2b ). Together with E-cadherin transcripts, other epithelial markers were also suppressed in CagA-positive 60190-infected gastric cancer cells, whereas mesenchymal markers increased ( Supplementary Fig. 2c ). The endogenous protein levels of other E-cadherin repressors such as Slug, Twist and Zeb1 were not detected regardless of H. pylori infection in AGS and MKN28 cells, nor was there significant change in Zeb2 protein levels ( Supplementary Fig. 2d ). Interestingly, CagA increased transfected Slug protein abundance ( Supplementary Fig. 2e ), suggesting that endogenous Snail plays a major role in the CagA-mediated EMT programme. 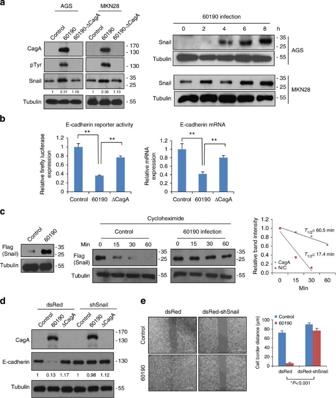Figure 2:H. pyloriCagA induces EMT through stabilization of Snail protein. (a) The CagA, endogenous Snail and phospho-Tyr (pTyr) levels were detected after treatment of 60190 or isogenic CagA deletion mutant strain (ΔCagA) in AGS and MKN28 cells (left panels). Relative protein abundance below the blot. Blots are representative of two independent experiments. The time-dependent abundances of Snail were determined by immunoblot analysis after infection with 60190 at the indicated time periods (right panels). Tubulin served as loading control. (b) E-cadherin proximal promoter activity (left panel) and E-cadherin transcript levels (right panel) were determined in 60190 or isogenic CagA deletion mutant strain in AGS cells. Activity of the E-cadherin promoter construct was normalized to the activity of the co-transfected SV-40renillaactivity. The relative abundance of E-cadherin transcripts in 60190 or CagA-deleted 60190 treated cells was compared with GAPDH. Relative reporter activity and mRNA abundance were determined from triplicate experiments (**P<0.01 by Student’st-test). Error bars indicate s.d. (c) Following the control or 60190 infections, Snail protein half-life was determined in AGS cells at the indicated time periods after treating the cycloheximide as described in Methods. The half-life of Snail was determined from the slope of densitometric protein abundance (right panel). (d) The Snail was stably knocked down with lentivirus in MKN28 cells (dsRed-shSnail), and the E-cadherin expression levels were detected by immunoblot analysis followed by CagA-positive 60190 infections or isogenic deletion strains for 24 h. Blots are representative of two independent experiments. (e) Confluent AGS cells of control dsRed and shRNA-mediated Snail knock-down cells were wounded using a pipette tip and then infected with control or 60190 strain for 4 h (left panels). Distance between cell borders was measured from five independent sites and the relative migratory inhibition by Snail knock-down compared with dsRed control cells was analysed using two-way analysis of variance test (right panel). Error bars indicate s.d. Figure 2: H. pylori CagA induces EMT through stabilization of Snail protein. ( a ) The CagA, endogenous Snail and phospho-Tyr (pTyr) levels were detected after treatment of 60190 or isogenic CagA deletion mutant strain (ΔCagA) in AGS and MKN28 cells (left panels). Relative protein abundance below the blot. Blots are representative of two independent experiments. The time-dependent abundances of Snail were determined by immunoblot analysis after infection with 60190 at the indicated time periods (right panels). Tubulin served as loading control. ( b ) E-cadherin proximal promoter activity (left panel) and E-cadherin transcript levels (right panel) were determined in 60190 or isogenic CagA deletion mutant strain in AGS cells. Activity of the E-cadherin promoter construct was normalized to the activity of the co-transfected SV-40 renilla activity. The relative abundance of E-cadherin transcripts in 60190 or CagA-deleted 60190 treated cells was compared with GAPDH. Relative reporter activity and mRNA abundance were determined from triplicate experiments (** P <0.01 by Student’s t -test). Error bars indicate s.d. ( c ) Following the control or 60190 infections, Snail protein half-life was determined in AGS cells at the indicated time periods after treating the cycloheximide as described in Methods. The half-life of Snail was determined from the slope of densitometric protein abundance (right panel). ( d ) The Snail was stably knocked down with lentivirus in MKN28 cells (dsRed-shSnail), and the E-cadherin expression levels were detected by immunoblot analysis followed by CagA-positive 60190 infections or isogenic deletion strains for 24 h. Blots are representative of two independent experiments. ( e ) Confluent AGS cells of control dsRed and shRNA-mediated Snail knock-down cells were wounded using a pipette tip and then infected with control or 60190 strain for 4 h (left panels). Distance between cell borders was measured from five independent sites and the relative migratory inhibition by Snail knock-down compared with dsRed control cells was analysed using two-way analysis of variance test (right panel). Error bars indicate s.d. Full size image Increased Snail protein half-life is an important regulatory mechanism of EMT [17] , [20] . To test whether CagA affects Snail stability, we transfected Flag-tagged Snail vector and chased Snail protein abundance under cycloheximide treatment. We found that the Snail protein half-life was significantly prolonged by 60190 infection compared with the negative control ( Fig. 2c ), suggesting that H. pylori CagA increases Snail protein abundance by prolonging the protein half-life. To further examine the influence of Snail on the CagA-induced EMT process, we made Snail knockdown cells with lentivirus-mediated small hairpin RNA (shRNA). When we compared E-cadherin expression under treatment of 60190, CagA translocation specifically suppressed E-cadherin expression in control cells, whereas Snail knockdown cells did not ( Fig. 2d and Supplementary Fig. 2f ). The migration potential of Snail knockdown cells was significantly decreased under 60190 infection ( Fig. 2e and Supplementary Fig. 3 ), indicating that Snail protein abundance plays an important role in the CagA-mediated EMT process. As CagA comprises multiple structural domains [29] , we next made several expression constructs to determine the domain of CagA responsible for stabilizing Snail ( Fig. 3a ). When we co-transfected the wt or phosphorylation-resistant (PR) mutant or deletion mutants of CagA with a minimum amount of Snail expression vector, Snail protein abundance was increased by all mutant constructs while innocuous green fluorescent protein (GFP) protein was unaffected ( Fig. 3b ). Intriguingly, the EPIYA phosphorylation motif on the C-terminus strongly reinforces CagA function on Snail abundance, whereas the N-terminus of CagA including domain I and a subdomain of domain II were only minimally or moderately effective [26] , [29] . These results indicate that multiple domains of CagA are responsible for the stabilization of Snail. 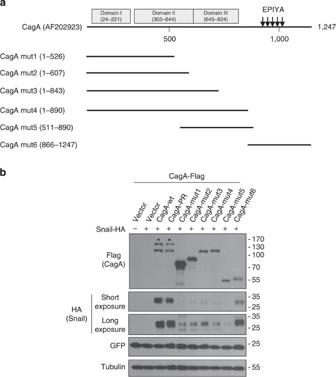Figure 3: Multiple domains of CagA are responsible for Snail protein stabilization. (a) Schematic diagram of Flag-tagged CagA expression vectors. Arrows indicate EPIYA phosphorylation on AF202923; structural domains of CagA with corresponding amino acid sequence are denoted by rectangular boxes29. (b) The wt or mutant CagA expression vectors were co-transfected with a minimum amount of Snail (50 ng) and GFP (200 ng) expression vectors in 293 cells for a 48 h period and the whole-cell lysates were subjected to immunoblot analysis. CagA-PR denotes tyrosine PR mutant on EPIYA motifs. *specific bands. Figure 3: Multiple domains of CagA are responsible for Snail protein stabilization. ( a ) Schematic diagram of Flag-tagged CagA expression vectors. Arrows indicate EPIYA phosphorylation on AF202923; structural domains of CagA with corresponding amino acid sequence are denoted by rectangular boxes [29] . ( b ) The wt or mutant CagA expression vectors were co-transfected with a minimum amount of Snail (50 ng) and GFP (200 ng) expression vectors in 293 cells for a 48 h period and the whole-cell lysates were subjected to immunoblot analysis. CagA-PR denotes tyrosine PR mutant on EPIYA motifs. *specific bands. Full size image CagA depletes GSK-3β activity in gastric cancer cells Because Snail protein stability was tightly controlled by GSK-3-mediated serial phosphorylation and subsequent proteasomal degradation [17] , [20] , we next examined GSK-3 levels and activities following 60190 infection into gastric cancer cells. Notably, translocation of CagA by H. pylori infection depleted the cellular GSK-3β as well as GSK-3α protein levels, accompanied by an increased insoluble fraction of CagA and GSK-3 ( Fig. 4a and Supplementary Fig. 4a ), suggesting that CagA transforms GSK-3 insoluble. The protein abundance of phospho-GSK-3β (Ser9), typical of inactive phosphorylation of GSK-3, decreased in tandem with total GSK-3. Given the ability of variable CagA expression to Snail protein abundance, we overexpressed CagA with HA-tagged GSK-3β to examine the transition of GSK-3β to insoluble fraction. Indeed, the expression of full-length or deletion mutants of CagA are enough to transform GSK-3 into insoluble fraction ( Fig. 4b ). Consistent with decreased abundance of soluble GSK-3, endogenous kinase activity was also attenuated by infection of H. pylori in both cells in a CagA-dependent manner ( Fig. 4c ). To examine whether CagA can bind to GSK-3β, the cells were infected with 60190 or an isogenic CagA deletion mutant strain and subjected to immunoprecipitation with GSK-3 antibody. Indeed, CagA was recovered from GSK-3β binding proteins ( Fig. 4d ). When we overexpressed flag-tagged CagA expression vector followed by immunoprecipitation with anti-flag agarose, endogenous GSK-3β including phospho-Ser9-GSK-3β was recovered from CagA ( Supplementary Fig. 4b ). To observe CagA and GSK-3 directly, we sought to determine the intracellular localization of CagA and GSK-3β by 60190 infections using immunofluorescence. As shown in Fig. 4e , CagA was co-localized with GSK-3β, especially in membranous localization, the cytosolic GSK-3 expression pattern changing to aggregate of various sizes following H. pylori infection. Though the transfection of CagA expression vector displayed a similar pattern ( Supplementary Fig. 4c ), the bacterial infection was more efficient for CagA protein abundance and aggregate formation with GSK-3. Further, 61090 infections dramatically increased the endogenous nuclear Snail level in the immunofluorescence study ( Fig. 4f ). Since the canonical Wnt suppresses GSK-3 activity through the sequestration of soluble GSK-3 in multivesicular endosomes [30] , we next examined the localization of CagA and Rab9, a GTPase of multivesicular body [31] . Interestingly, the localization of CagA and endogenous Rab9 was mutually exclusive in cells ( Supplementary Fig. 5a ), demonstrating that endogenous Rab9 was mainly localized in perinuclear cytosolic spaces, whereas exogenous CagA was in juxtamembranous portion. These results indicate that inactivation of GSK-3 by CagA is independent of multivesicular endosomes. 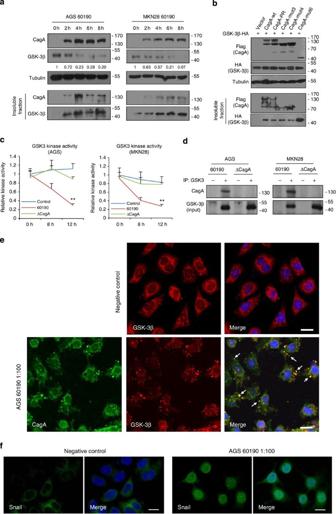Figure 4: CagA binds and depletes endogenous GSK-3. (a) Following the infection with 61090, time-course protein abundances of CagA and GSK-3β in Triton X-100-soluble or insoluble fractions were determined by immunoblot analysis in cells. Note the decrease in GSK-3β protein abundance of soluble fraction in a time-dependent manner. Tubulin was used as the loading control. (b) The wt or mutant CagA expression vectors were co-transfected with a HA-tagged GSK-3β expression vector in 293 cells for a 48 h period. The transition of GSK-3β into insoluble fractions was detected by immunoblot analysis against anti-HA antibody. (c) The endogenous GSK-3 kinase activity in AGS and MKN28 cells was measured. The samples from 0 h, 8 h and 12 h with time-course negative control were subjected to the kinase assay following infection with 60190 or CagA-deleted 60190 (ΔCagA), or with untreated control. The relative kinase activity was determined from triplicate experiments. **P<0.01 compared with control and to ΔCagA treatment by Student’st-test. Error bars indicate s.d. (d) The AGS and MKN28 cells were infected with control or 60190 or CagA-deleted 60190 (ΔCagA) for 2 h. The GSK-3–CagA complexes were isolated in immunoprecipitates recovered from the lysates following pull-down with anti-GSK-3β monoclonal antibody and immunoblot with anti-CagA or polyclonal GSK-3β antibody. Mouse IgG was used for negative control (–) of anti-GSK-3β antibody. (e) AGS cells were transfected with HA-tagged GSK-3β expression vector in combination with control (upper panels) or 60190 infections (lower panels). The cells were stained with anti-CagA (green) and anti-HA to localize GSK-3β (red), and DAPI to visualize nuclei (blue) by confocal microscopy. White arrows in the merged image indicate co-localized membranous GSK-3 and CagA. Scale bar, 20 μm. (f) AGS cells were infected with negative control (left panels) or 60190 (right panels) and endogenous Snail was detected by immunofluorescence (green). Scale bar, 20 μm. Figure 4: CagA binds and depletes endogenous GSK-3. ( a ) Following the infection with 61090, time-course protein abundances of CagA and GSK-3β in Triton X-100-soluble or insoluble fractions were determined by immunoblot analysis in cells. Note the decrease in GSK-3β protein abundance of soluble fraction in a time-dependent manner. Tubulin was used as the loading control. ( b ) The wt or mutant CagA expression vectors were co-transfected with a HA-tagged GSK-3β expression vector in 293 cells for a 48 h period. The transition of GSK-3β into insoluble fractions was detected by immunoblot analysis against anti-HA antibody. ( c ) The endogenous GSK-3 kinase activity in AGS and MKN28 cells was measured. The samples from 0 h, 8 h and 12 h with time-course negative control were subjected to the kinase assay following infection with 60190 or CagA-deleted 60190 (ΔCagA), or with untreated control. The relative kinase activity was determined from triplicate experiments. ** P <0.01 compared with control and to ΔCagA treatment by Student’s t -test. Error bars indicate s.d. ( d ) The AGS and MKN28 cells were infected with control or 60190 or CagA-deleted 60190 (ΔCagA) for 2 h. The GSK-3–CagA complexes were isolated in immunoprecipitates recovered from the lysates following pull-down with anti-GSK-3β monoclonal antibody and immunoblot with anti-CagA or polyclonal GSK-3β antibody. Mouse IgG was used for negative control (–) of anti-GSK-3β antibody. ( e ) AGS cells were transfected with HA-tagged GSK-3β expression vector in combination with control (upper panels) or 60190 infections (lower panels). The cells were stained with anti-CagA (green) and anti-HA to localize GSK-3β (red), and DAPI to visualize nuclei (blue) by confocal microscopy. White arrows in the merged image indicate co-localized membranous GSK-3 and CagA. Scale bar, 20 μm. ( f ) AGS cells were infected with negative control (left panels) or 60190 (right panels) and endogenous Snail was detected by immunofluorescence (green). Scale bar, 20 μm. Full size image Consequences of GSK-3 depletion on oncogenic pathways To obtain evidence of GSK-3 phosphorylation on Snail, we chose a PR mutant of Snail [17] . When we co-expressed Snail vectors with CagA, GSK-3 PR Snail (Ser104,107Ala mutant) was minimally affected, whereas the wt Snail abundance was significantly increased ( Fig. 5a ). Because the anti-phospho-β-catenin antibody can detect GSK-3-dependent phospho-Snail due to its conserved sequence identity [17] , [32] , we used this antibody to determine whether CagA inhibits GSK-3-dependent phosphorylation of Snail. Indeed, the phosphorylation of Snail in semiquantitated immunoprecipitated samples was markedly suppressed by CagA ( Fig. 5b ), indicating that CagA increases Snail protein abundance through inhibition of phosphorylation. 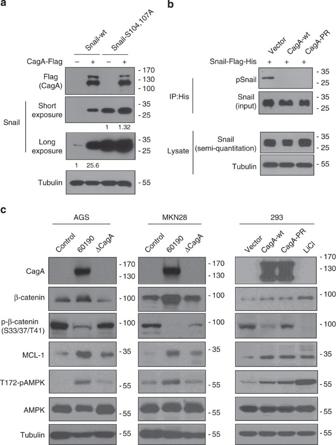Figure 5: The consequences of GSK-3 downregulation on Snail and other oncogenic pathways. (a) Flag-tagged wt Snail and PR mutant (S104,107A) were co-transfected with full-length CagA in 293 cells. The Snail protein abundance was detected with immunoblot analysis against anti-Flag antibody. Relative protein abundance of each loading control is denoted below the blots. (b) Flag-His-tagged wt Snail was co-transfected with control or CagA expression vector for 48 h. GSK-3-mediated phosphorylated Snail was determined following immunoprecipitation (1 × , 1/3 × , 1/3 × volume of the respective cell lysate for Snail semi-quantitation) with minimum amount of Ni-Ti beads to saturate protein binding and, subsequent immunoblot analysis with anti-phospho-β-catenin antibody (pSnail). (c) The abundance of GSK-3β regulated proteins, total β-catenin, phospho-β-catenin (S33/37/T41), MCL-1, T172-phospho-AMPK and total AMPK were detected after infection with control or 60190 or isogenic CagA deletion mutant strain (ΔCagA) in AGS and MKN28 cells (left and middle panels). The 293 cells transfected with control or full-length of wt CagA or PR mutant CagA were subjected to the same panel of antibodies (right panels). As a control of GSK-3 inhibition, the 40 mM of LiCl were treated for 3 h before protein harvest. Figure 5: The consequences of GSK-3 downregulation on Snail and other oncogenic pathways. ( a ) Flag-tagged wt Snail and PR mutant (S104,107A) were co-transfected with full-length CagA in 293 cells. The Snail protein abundance was detected with immunoblot analysis against anti-Flag antibody. Relative protein abundance of each loading control is denoted below the blots. ( b ) Flag-His-tagged wt Snail was co-transfected with control or CagA expression vector for 48 h. GSK-3-mediated phosphorylated Snail was determined following immunoprecipitation (1 × , 1/3 × , 1/3 × volume of the respective cell lysate for Snail semi-quantitation) with minimum amount of Ni-Ti beads to saturate protein binding and, subsequent immunoblot analysis with anti-phospho-β-catenin antibody (pSnail). ( c ) The abundance of GSK-3β regulated proteins, total β-catenin, phospho-β-catenin (S33/37/T41), MCL-1, T172-phospho-AMPK and total AMPK were detected after infection with control or 60190 or isogenic CagA deletion mutant strain (ΔCagA) in AGS and MKN28 cells (left and middle panels). The 293 cells transfected with control or full-length of wt CagA or PR mutant CagA were subjected to the same panel of antibodies (right panels). As a control of GSK-3 inhibition, the 40 mM of LiCl were treated for 3 h before protein harvest. Full size image GSK-3 is highly active under resting state and numerous substrates of GSK-3 have been identified in a wide range of cellular processes [33] . To extend our observations to other oncogenic pathways, we next examined the antiapoptotic BCL-2 family member, MCL-1, which harbours the canonical GSK-3 phosphorylation motif responsible for the subsequent β-TrCP-mediated degradation process similarly to β-catenin and Snail [34] , [35] . Recently, the AMPK catalytic subunit has also been identified as an atypical substrate of GSK-3, whereby GSK-3 inhibits Thr172 phosphorylation of AMPK-α and its catalytic activity [36] . When we infected cells with 60190 or overexpressed CagA, total β-catenin protein abundance increased; in contrast, amino-terminal (N-terminal) phosphorylation of β-catenin was decreased ( Fig. 5c ). The MCL-1 protein abundance and phosphorylation of Thr172 of AMPK-α were significantly potentiated by CagA transduction, indicating that functional consequences of CagA-mediated depletion of GSK-3 comprise a wider spectrum of oncogenic pathways. The EPIYA region on CagA binds to GSK-3β The carboxyl-terminal (C-terminal) region of CagA is mainly responsible for morphological changes in epithelial cells [26] , [37] , whereas the tyrosine phosphorylation on the EPIYA motif contributes to the cytoskeletal rearrangement and cell elongation. Given the ability of full-length CagA to bind to GSK-3, we made GFP-Flag-fusion constructs having EPIYA motifs and co-transfected them with GSK-3β expression vector to further determine the role of the EPIYA region ( Fig. 6a ). Indeed, GFP fusion proteins having EPIYA motifs were able to bind GSK-3β, while the proximal region of EPIYA was not ( Fig. 6b ). During the Wnt signal transduction, Axins serve as scaffolding proteins that interact with GSK-3β and act as regulators of its subcellular localization and kinase activity [18] . In this process, the phosphorylation of Tyr216 and conformational plasticity of the C-terminal loop in GSK-3β provide a binding site for Axin [18] , [19] , [38] . To test whether EPIYA motif on CagA shares a similar binding site with Axin, we selected GSK-3β mutant Val267/Glu268 (rendered unable to bind Axin by disturbing ridge–groove interactions) and mutant Tyr216 (refs 18 , 20 ). When we examined interactions between GFP-EPIYA construct and GSK-3β mutants, the EPIYA on CagA was not bound to C-terminal loop mutants of GSK-3β similarly to Axin though the binding was independent of Tyr216 phosphorylation ( Fig. 6c ). Consistent with this finding, mutant Val267/Glu268 was not insolubilized by CagA compared with wt GSK-3 ( Supplementary Fig. 5b ). Because N-terminal phosphorylation of GSK-3 (Ser9 of GSK-3β) is well known to inactivate GSK-3, we next used an N-terminal deletion mutant (Δ9-GSK-3β) to examine whether this phosphorylation is involved in CagA binding. Interestingly, CagA bound to GSK-3β regardless of N-terminal deletion ( Fig. 6d ). To further examine GSK-3 binding to CagA in a mammalian cell free system, we subjected bacterial lysates to immunoprecipitation study with recombinant GSK-3β followed by competitive elution with synthetic Axin peptide (aa 383–401) [19] . Intriguingly, the CagA protein was recovered by Axin peptide competition ( Fig. 6e ). These results provide additional evidence that the binding of CagA and GSK-3 is important for H. pyroli -mediated GSK-3 depletion resulting in the activation of the EMT programme and other oncogenic pathways ( Fig. 6f ). 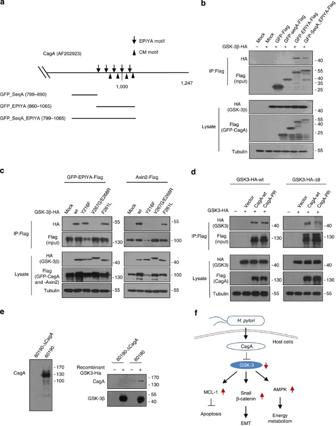Figure 6: C-terminus of CagA binds to GSK-3β through the Axin binding site. (a) Schematic diagram of GFP-Flag-fusion constructs for CagA C-terminus. Arrows and arrowheads denote EPIYA and multimerization domain on AF202923, respectively. (b) The 293 cells were either transfected with control or with Flag-tagged GFP-fusion constructs as indicated in combination with HA-tagged GSK-3β expression vector for a 48 h period. The GSK-3β binding affinity of GFP-CagA fusion constructs was detected by immunoprecipitation with anti-Flag agarose following immunoblot analysis with either anti-Flag (GFP-CagA) or anti-HA (GSK-3β) antibody. (c) The Flag-tagged GFP-EPIYA fusion constructs or Axin2 were co-transfected with various types of HA-GSK-3β mutant in 293 cells as indicated for 48 h. The lysates were subjected to immunoprecipitation with anti-Flag agarose and the GSK-3β binding ability to CagA or Axin2 was detected with immunoblot analysis. (d) The wt or mutant CagA expression vectors were co-transfected with a HA-tagged GSK-3β (wt) or N-terminal deleted GSK-3β (Δ9) expression vector in 293 cells. The binding affinity of GSK-3β to CagA was assessed by immunoprecipitation with anti-flag agarose and immunoblot analysis against anti-HA antibody. (e) Immunoblot analysis of bacterial CagA protein in 60190 or ΔCagA strain (left panel). His-tagged recombinant GSK-3β from sf9 insect cell was incubated with bacterial lysates of 60190 or ΔCagA strain for 1 h, followed by 100 ng of Axin peptide competition on GSK-3 binding. The eluted CagA and GSK-3β on Ni-Ti beads were detected by immunoblot analysis (right panels). (f) Schematic diagram of CagA-mediated GSK-3 depletion and subsequent activation of EMT and other oncogenic pathways. Following transduction of CagA into the cells via a type IV secretion system, the cytoplasmic GSK-3 is rapidly insolubilized and downregulated, resulting in the activation of the GSK-3-dependent oncogenic pathway. Figure 6: C-terminus of CagA binds to GSK-3β through the Axin binding site. ( a ) Schematic diagram of GFP-Flag-fusion constructs for CagA C-terminus. Arrows and arrowheads denote EPIYA and multimerization domain on AF202923, respectively. ( b ) The 293 cells were either transfected with control or with Flag-tagged GFP-fusion constructs as indicated in combination with HA-tagged GSK-3β expression vector for a 48 h period. The GSK-3β binding affinity of GFP-CagA fusion constructs was detected by immunoprecipitation with anti-Flag agarose following immunoblot analysis with either anti-Flag (GFP-CagA) or anti-HA (GSK-3β) antibody. ( c ) The Flag-tagged GFP-EPIYA fusion constructs or Axin2 were co-transfected with various types of HA-GSK-3β mutant in 293 cells as indicated for 48 h. The lysates were subjected to immunoprecipitation with anti-Flag agarose and the GSK-3β binding ability to CagA or Axin2 was detected with immunoblot analysis. ( d ) The wt or mutant CagA expression vectors were co-transfected with a HA-tagged GSK-3β (wt) or N-terminal deleted GSK-3β (Δ9) expression vector in 293 cells. The binding affinity of GSK-3β to CagA was assessed by immunoprecipitation with anti-flag agarose and immunoblot analysis against anti-HA antibody. ( e ) Immunoblot analysis of bacterial CagA protein in 60190 or ΔCagA strain (left panel). His-tagged recombinant GSK-3β from sf9 insect cell was incubated with bacterial lysates of 60190 or ΔCagA strain for 1 h, followed by 100 ng of Axin peptide competition on GSK-3 binding. The eluted CagA and GSK-3β on Ni-Ti beads were detected by immunoblot analysis (right panels). ( f ) Schematic diagram of CagA-mediated GSK-3 depletion and subsequent activation of EMT and other oncogenic pathways. Following transduction of CagA into the cells via a type IV secretion system, the cytoplasmic GSK-3 is rapidly insolubilized and downregulated, resulting in the activation of the GSK-3-dependent oncogenic pathway. Full size image H. pylori infection increases Snail in clinical samples Given the ability of H. pylori CagA to induce Snail stabilization, we sought to determine whether H. pylori infection drives Snail expression in gastric tissue. We chose endoscopic biopsy samples from patients diagnosed as non-specific or H. pylori gastritis (eight cases each group) and assessed Snail protein abundance in gastric epithelium by immunohistochemistry. Indeed, the Snail protein abundance in nuclei was higher in H. pylori gastritis epithelium ( Fig. 7a and Supplementary Fig. 6 ). The relative nuclear staining intensity of epithelial cells compared with endothelial cells supports that H. pylori infection potentiates Snail expression in human gastric epithelium ( Fig. 7b ). 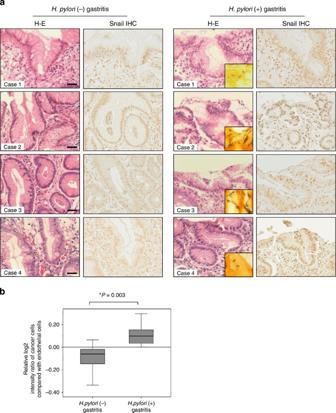Figure 7:H. pyloriinfection potentiates Snail abundance in clinical samples. (a) Routine H/E section and Snail expression detected by immunohistochemistry inH. pylori(−) or (+) gastritis samples from endoscopic biopsy.H. pyloriinfection on gastric epithelium was validated with Warthin–Starry staining (insets). Scale bar, 100 μm. Digital images of immunostaining were taken with Aperio Scanscope. See alsoSupplementary Fig. 5for additional cases. (b) Relative Snail staining intensity of epithelial cells to endothelial cells was determined by image analysis as described in the Methods. The relative log expression values were represented and the statistical difference was obtained using the Student’st-test. Box plots represent the median (horizontal line) and interquartile range (box) of the indicated distribution. The whiskers extend from the top/bottom of the box to the highest/lowest data value. Figure 7: H. pylori infection potentiates Snail abundance in clinical samples. ( a ) Routine H/E section and Snail expression detected by immunohistochemistry in H. pylori (−) or (+) gastritis samples from endoscopic biopsy. H. pylori infection on gastric epithelium was validated with Warthin–Starry staining (insets). Scale bar, 100 μm. Digital images of immunostaining were taken with Aperio Scanscope. See also Supplementary Fig. 5 for additional cases. ( b ) Relative Snail staining intensity of epithelial cells to endothelial cells was determined by image analysis as described in the Methods. The relative log expression values were represented and the statistical difference was obtained using the Student’s t -test. Box plots represent the median (horizontal line) and interquartile range (box) of the indicated distribution. The whiskers extend from the top/bottom of the box to the highest/lowest data value. Full size image Loss of epithelial adhesion, a hallmark of EMT, constitutes a part of the genetic background of hereditary and sporadic gastric adenocarcinoma [13] , [14] ; transcriptional repressor Snail is a well-known EMT inducer, which suppresses E-cadherin transcription [15] . In addition to mutational inactivation, polymorphism and hypermethylation on the proximal promoter of E-cadherin also lead to silencing of E-cadherin in gastric cancer cells [39] , [40] , [41] . Although EMT is typically observed in the invasive progression of cancer, in vivo evidence suggests that loss of epithelial adhesion is sufficient to initiate invasive adenocarcinoma in pancreas and stomach [40] , [42] and inducible expression of Snail leads to irreversible tumorigenesis in mice [27] . Interestingly, systemic expressions of CagA and Snail in vivo share similar phenotypic outcomes of haematopoietic malignancies [9] , [27] . GSK-3 is highly expressed and is one of the few kinases inactivated following stimulation of exogenous signalling. For example, Wnt signalling suppresses cytosolic GSK-3 activity through the sequestration of GSK-3 from the cytosol into acidic multivesicular bodies [30] . On the other hand, the growth factors, insulin or treatment of serum rapidly inhibits GSK-3 activity via N-terminal phosphorylation (of Ser21 for GSK-3α and Ser9 for GSK-3β) while the phosphorylation is independent of Axin function in Wnt [20] . We found that bacterial CagA translocation rapidly inactivated both forms of GSK-3α and GSK-3β within a few hours. Among a wide variety of GSK-3 substrates, Snail, β-catenin, and MCL-1 harbour the typical GSK-3β phosphorylation serial motif governing the EMT process and an antiapoptotic function [17] , [20] , [34] , [35] . Further, the catalytic function of AMPK-α is also inhibited by GSK-3 through an atypical phosphorylation motif [36] . In this study, we showed that the inhibition of GSK-3 activity by CagA significantly increases the protein abundance of MCL-1 and catalytically active AMPK as well as of Snail. These results demonstrate that the depletion of GSK-3 by H. pylori CagA translocation comprises a wide range of oncogenic pathways beyond the activation of Wnt signalling and the EMT programme. CagA, a 120–145 kDa protein, interacts with many proteins to activate intracellular signalling [5] . EMT-like morphogenetic changes accompanying cytoskeletal rearrangement by CagA, known as the ‘hummingbird phenotype’, have been noted in epithelial cells, similar to changes due to the scatter factor of HGF (hepatocyte growth factor) [24] . While the CagA expression vector has allowed versatile protein interaction studies, translocation of CagA through the bacterial type IV secretion system was more efficient in terms of GSK-3 depletion in cells. Further study is required to determine the importance of other virulence factors, such as VacA and intracellular delivery of peptidoglycan, in bacterial CagA functions [1] , [2] . The C-terminal region of CagA provides a binding site for SHP2 and PAR1/MARK2 following EPIYA phosphorylation and phenotypic transformation [3] , [10] , [43] . Importantly, CagA perturbs the E-cadherin/β-catenin complex, resulting in the accumulation of cytoplasmic and nuclear β-catenin [44] . In this process, the multimerization sequence embedded in EPIYA-repeats is responsible for E-cadherin binding, β-catenin activation and acquisition of the EMT phenotype [26] , [44] , [45] . Consistent with previous findings that the EPIYA repeated region is responsible for the activation of β-catenin [45] , we found that a C-terminal region having an EPIYIA and multimerization domain plays an important role in binding to and depletion of GSK-3. Intriguingly, GSK-3 can phosphorylate PAR1/MARK2, which is responsible for tau phosphorylation in Alzheimer disease [46] . The tertiary structure of CagA, consisting of N-terminal structured domains and a disordered C-terminal region, indicates that EPIYA motif phosphorylation plays important roles in entire CagA structure and protein interactions [29] . In this study, we found that multiple domains of CagA are also responsible for Snail stabilization and that the C-terminus of CagA having the EPIYA motif binds to GSK-3 (refs 19 , 38 ). Considering that a dynamic CagA structure having α-helices and undergoing activation of the Wnt/EMT process depends on more than EPIYA phosphorylation [26] , [29] , [45] , it is not surprising that many domains of CagA are able to bind GSK-3, resulting in depletion of GSK-3 and subsequent increased Snail protein abundance. Protein binding between Axin and GSK-3 is required to activate the intracellular cascade of Wnt signalling and the Snail-mediated EMT programme via regulation of membranous and nuclear-cytosolic dynamics [20] , [47] . Notably, p53 tumour suppressor regulates nuclear GSK-3β activity through miRNA-34-mediated Axin2 suppression in colorectal cancers [48] , implying that the intracellular dynamics and kinase activity of GSK-3 play an important role in carcinogenesis. Interestingly, Kaposi’s sarcoma-associated herpes virus-encoded latency-associated nuclear antigen (LANA) also binds to GSK-3 similarly to Axin, resulting in suppression of GSK-3 activity [49] , [50] , [51] . Thus, pathogenic gene products of microbes may commonly target GSK-3 with an Axin/CagA binding site, resulting in the activation of oncogenic pathways coupled with the Snail-mediated EMT programme. Colonization by the CagA-positive H. pylori strain induces both acute and chronic inflammation in the superficial epithelium of host stomach. Although the induction of inflammatory cytokine secretion and activation of signalling pathways by CagA have been demonstrated [52] , the molecular mechanism of the inflammatory response due to CagA has not yet been clearly defined. Although Snail has been found to induce EMT during cancer invasion and metastasis [15] , recent evidence suggests that increased Snail abundance in epithelial cells significantly upregulates cyclooxygase-2 and proinflammatory cytokines such as interleukin-8 (IL-8), IL-1 and IL-6, accompanied by acquisition of an invasive phenotype [53] . Furthermore, the prolonged expression of Snail in epidermal keratinocytes is sufficient to induce cutaneous inflammation in mice [54] . Our results thus imply that Snail stabilization by CagA may constitute a molecular link in H. pylori -mediated inflammation as well as in carcinogenesis in gastric epithelial cells. Further detailed structural characterization of CagA is required to understand variable pathogenicity of H. pylori strains in terms of GSK-3 depletion, inflammatory response and activation of oncogenic pathways. Bacteria, cell culture and co-culture with H. pylori H. pylori strains 60190 (ATCC 49503, cag PAI+) and Δ CagA (an isogenic mutant of 60190 lacking CagA ) were used as described previously [8] . Briefly, H. pylori strains were cultured on blood agar plates containing 5% horse serum at 37 °C in a microaerobic atmosphere using the Campy Container System (BBL, Sparks, MD). Human gastric epithelial cells (AGS, MKN28) and 293 cells obtained from American Type Culture Collection were routinely cultured in RPMI 1640 and Dulbecco’s Modified Eagle’s medium containing 10% fetal bovine serum. When gastric epithelial cells reached 70% confluence, they were serum-starved overnight before addition of H. pylori at a multiplicity of infection of 30. Expression vectors and immunoblot analysis Full-length constructs for CagA (AF202923) and PR mutant on EPIYA were kindly provided by Professor M. Hatakeyama. The full-length or deletion mutant CagA expression constructs were cloned into pCMV-3xFlag expression vectors (Sigma) using a PCR-based technique. The Flag-His- or HA-tagged human Snail, Slug, HA-tagged GSK-3β, HA-tagged N-terminal deletion GSK-3 β (aa 1–9) expression vectors and wt and E-box mutated E-cadherin proximal promoter reporters were used as described previously [17] , [20] . Briefly, the C-terminal Flag-His or HA-tagged human cDNA of Snail and Slug were subcloned into pCR3.1 (Invitrogen) mammalian expression vector. HA-tagged human GSK-3β was obtained from Addgene (plasmid number 14753). An expression vector for EPIYA domain fused with GFP or GSK-3β mutants were generated with PCR-based methods. shRNA expression construct for Snail and lentiviral transduction were performed as described previously [20] , [23] . Immunoblot analysis with Triton X-100 lysate was performed as described previously [17] , [20] . Briefly, the insoluble pellets from Triton X-100 lysis buffer were re-suspended in SDS-RIPA buffer followed by heating at 95 °C for 5 min and high-speed centrifugation. The relative band intensity of protein abundance compared with loading control in immunoblot analysis was quantified by densitometer and the relative value was denoted below the blot as indicated. The commercially available primary antibodies were directed against Snail (1:1,000 for IB, Cell Signaling 3896S), rabbit anti-CagA (1:5,000, Ostral HPP-5003-9), mouse monoclonal anti-GSK-3β (1:2,500, BD Bioscience 610202), rabbit polyclonal anti-GSK-3β (1:500, Santa Cruz sc-9166), anti-GSK-3 (1:1,000, Abcam ab82542), anti-phospho-Tyr (1:1,000, Santa Cruz sc-7020), E-cadherin (1:5,000, BD Bioscience 610181), Twist (1:500, Abgent AT4410a), Slug (1:1,000, Cell Signaling 9585S), Zeb1 (1:1,000, Cell Signaling 3396S), Zeb2 (1:500, Abgent AT4573a), mouse anti-HA (1:1,000, Roche 11583816001), rabbit anti-HA (1:500, Clontech 631207), anti-Rab-9 (1:500, Cell Signaling 2095), anti-MCL-1 (1:2,000, Santa Cruz sc-819), anti-phosphoThr172-AMPK (1:1,000, Cell Signaling 2535S), anti-AMPK (1:1,000, Cell Signaling 2793S), anti-phospho-β-catenin (S33/37/T41; 1:1,000, Cell Signaling 9561) and anti-Flag-M2 (1:5,000, Sigma F3165). The rabbit polyclonal antibody against Snail was described previously [20] . For immunoprecipitation analysis, whole-cell Triton X-100 lysates were incubated with Flag-M2 agarose (Sigma) or protein G agarose (Invitrogen). The recovered proteins of 1/20 volume for input were resolved by SDS-PAGE and subjected to immunoblot analysis. His-tagged recombinant GSK-3β from sf9 insect cells was kindly provided by Professor Hyun Soo Cho (Yonsei University). The 19-mer Axin peptide (Axin1, aa 383–401, VEPQKFAEELIHRLEAVQR), which is known to bind GSK-3 as an amphipathic α-helix, was chemically synthesized (Peptron) [19] . The bacterial lysate of 60190 and CagA-deleted 60190 were prepared from Triton X-100 lysis buffer, and the lysates were subjected in Ni-Ti beads (Invitrogen) with His-tagged recombinant GSK-3 to examine direct binding between CagA and recombinant GSK-3β. The CagA bound to GSK-3 was eluted by adding 100 ng of Auxin peptide, and the elution samples were subject to immunoblot analysis with CagA antibody. The pulse-chase analyses of Snail were performed as described previously [23] , followed by infection of 60190 in AGS cells. Whole-blot images are presented in Supplementary Fig. 7 . Quantitative real-time RT-PCR Total RNA was prepared using TRIZOL (Invitrogen) following the manufacturer’s protocol and quantitative real-time reverse transcriptase–PCR (RT-PCR) was performed as described previously [22] . Briefly, the cDNAs were generated from 1 μg of total RNA using Superscript II reverse transcriptase (Invitrogen) and random hexamer primer according to the recommendations of the manufacturer. Quantitative real-time RT-PCR was performed using specific sense and antisense primers ( Supplementary Table 1 ) in a 10 μl reaction volume containing 5 ul of Applied Biosystems 2X SYBR Green Mix, 0.25 pmol of each primer and 100 ng of cDNA. Real-time PCR was performed using the Applied Biosystems STEP One detection system. The expression of Δ C t value from each sample was calculated by normalizing with GAPDH from triplicate experiment. Immunofluorescence study Cells were washed twice with ice-cold PBS and incubated for 15 min at room temperature with 3% formaldehyde in PBS. The cells were permeabilized with 0.5% Triton X-100 for 5 min and then blocked for 1 h in PBS containing 3% bovine serum albumin and incubated with primary antibody overnight at 4 °C. Cells were then washed several times with PBS containing 0.1% Tween 20 followed by incubation with anti-mouse-FITC- and/or anti-rabbit-Texas Red-conjugated secondary antibody, then DAPI for 1 h at room temperature with PBST washing. Cellular fluorescence was monitored using confocal microscopy (Zeiss). GSK-3β kinase assay The GSK-3β kinase activity assay from cell lysate was performed using the GSK-3β kinase assay kit (ENZO Biochem Inc.) according to the manufacturer’s instructions. Reporter gene assay AGS or MKN28 cells were co-transfected with 0.1 μg of reporter gene construct E-cadherin (−108) or 3 × E-box mutants with 2 ng of pSV-40 renilla 24 h before H. pylori infection. The reporter activities were measured with a dual luciferase assay kit (Promega) 24 h after infection of 60190 or isogenic strain of CagA deletion, then normalized with renilla activities. Reporter activities were presented as relative light units to those obtained from the negative control. The results are expressed as the averages of the ratios of the reporter activities from triplicate experiments. Invasion and migration assay Invasive activity of gastric cancer cells was determined using a matrigel-coated transwell chamber system with an 8μm-pore polycarbonate membrane (Costar Corning, Acton, MA, USA) as described previously [16] , [23] . Briefly, the gastric epithelial cell lines were seeded on the top of the matrigel in the upper chamber while the bottom chambers were filled with regular culture medium. After 24 h incubation of the transwell system at 37 °C, the cells that had migrated through the membrane were fixed with Diff-Quik fixative (Sysmex), stained with Diff-Quik solution, and counted from five independent sites. For cell migration assays, confluent monolayers of AGS cells were wounded using pipette tip. After washing with culture medium twice to remove cell debris, cells were infected with H. pylori at a MOI of 30. For transient expression with vector, the cells were transfected with CagA expression vector before 24 h of migration assay. Wound closure was examined by light microscopy and the vertical distances between cell borders were represented as averages from five scratched sites. Cancer cell invasion of MCF-7 cells into the live CAM of 11-day-old chick embryos was performed as described previously [20] . Briefly, the cells were transiently co-transfected with GFP vector and control empty vector, or p3x-flag-CagA expression vector, before 24 h CAM invasion assay. The invasion was monitored after a 3-day culture period in cross sections of the fixed CAM by fluorescent microscopy from three independent experiments. GFP-positive cells were quantitated as invasive cancer cells under 10 high power fields for statistical analysis. Clinical gastric tissue samples and immunohistochemistry The paraffin-embedded specimens were obtained from endoscopic samples diagnosed with gastritis, including eight cases each of gastritis by non-specific inflammation or H. pylori infection. All specimens were provided by the Gastrointestinal Tumor Working Group Tissue Bank, Yonsei University Medical Center. The study protocol and exemption of informed consent were approved by the Institutional Review Board of the Severance Hospital in Yonsei Health System (4-2010-0265). For histological and immunohistochemical examination, serial paraffin sections were stained with haematoxylin and eosin for routine morphological observation and the H. pyroli infection was validated with Warthin–Starry stain. For immunohistochemical study of Snail, tissue sections in microslides were deparaffinized with xylene, hydrated in serial dilutions of alcohol, and immersed in 3% H 2 O 2 . Following antigen retrieval in citrate buffer (pH 6.0), the tissue sections were incubated with protein blocking agent for 20 min at room temperature and then incubated overnight at 4 °C with primary antibody (1:500) against Snail. After washing with PBS three times, the sections were incubated with a biotinylated secondary antibody (Immunotech) and streptavidin conjugated to horseradish peroxidase (Immunotech) for 20 min at room temperature, followed by a PBS wash. The chromogen was developed for 5 min with 3-amino-9-ethylcarbazole (AEC) followed by counterstain with Meyer’s haematoxylin. Image analysis was performed to quantify the Snail immunostaining intensity. Briefly, digital images of stomach epithelial cells (more than 100 cells each) were taken and colour saturation intensity was obtained. To avoid colour variation among samples, the images of endothelial cells in the same samples were taken simultaneously as an internal control. The log2 value of staining intensity of Snail in epithelial cells relative to endothelial cells was calculated. Statistical analysis Data from reporter, quantitative RT-PCR, migration and kinase assay were analysed using Student’s t -test. The double asterisks denote P <0.01, one asterisk denotes P <0.05. Statistical analysis for relative migration of dsRed and dsRed-shSnail cells following 60190 infection was performed using two-way analysis of variance test. How to cite this article: Lee, D.-G. et al . Helicobacter pylori CagA promotes Snail-mediated epithelial–mesenchymal transition by reducing GSK-3 activity. Nat. Commun. 5:4423 doi: 10.1038/ncomms5423 (2014).